miR-508 sustains phosphoinositide signalling and promotes aggressive phenotype of oesophageal squamous cell carcinoma The strength and duration of phosphoinositide signalling from phosphatidylinositol-3-kinase (PI3K) activation to Akt is tightly balanced by phosphoinositide kinases and phosphatases. However, how phosphatase-mediated negative regulatory effects are concomitantly disrupted in cancers, which commonly exhibit constitutively activated PI3K/Akt signalling, remains undefined. Here we report that miR-508 directly suppresses multiple phosphatases, including inositol polyphosphate-5-phosphatase J (INPP5J), phosphatase and tensin homologue (PTEN) and inositol polyphosphate 4-phosphatase type I (INPP4A), resulting in constitutive activation of PI3K/Akt signalling. Furthermore, we find that overexpressing miR-508 promotes, while silencing miR-508 impairs, the aggressive phenotype of oesophageal squamous cell carcinoma (ESCC) both in vitro and in vivo . Importantly, the level of miR-508 correlates with poor survival and activated PI3K/Akt signalling in a large cohort of ESCC specimens. These findings uncover a mechanism for constitutive PI3K/Akt activation in ESCC, and support a functionally and clinically relevant epigenetic mechanism in cancer progression. Phosphoinositides, the polyphosphorylated derivatives of phosphatidylinositol (PI), are membrane-bound signalling molecules that have crucial roles in most, if not all, cellular processes [1] , [2] , [3] . Under physiological conditions, the strength and duration of phosphoinositide signalling from phosphatidylinositol-3-kinase (PI3K) activation to Akt (protein kinase B) is tightly balanced both spatially and temporally by subcellularly localized PI kinases and phosphatases [4] , [5] . For instance, phosphatidylinositol-3,4-bisphosphate [PI(3,4)P2] and phosphatidylinositol -3,4,5-trisphosphate [PI(3,4,5)P3], phosphorylated by PI3K at the 3 position hydroxyl group of the inositol ring of PI, directly associate with Akt and phosphoinositide-dependent kinases through their pleckstrin homology domains, leading to activation of Akt kinase by two phosphorylation events at Thr 308 and Ser 473 (refs 4 , 6 , 7 ). The activated Akt further phosphorylates multiple downstream effectors, such as glycogen synthase kinase-3 (GSK3α/β), tuberous sclerosis complex-2 and FoxO-family transcription factors, together providing potent growth, proliferation, survival and anti-apoptotic signals to the cells [8] , [9] , [10] . On the other hand, the intracellular level of PI (3,4,5) P3 is negatively regulated by inositol polyphosphate 3-phosphatase or inositol polyphosphate 5-phosphatases [1] . For instance, the inositol polyphosphate 3-phosphatase PTEN (phosphatase and tensin homologue) dephosphorylates the 3 position of PI(3,4,5)P3 to generate PI(4,5)P2, and the 5-phosphatases, such as inositol polyphosphate-5-phosphatase J (INPP5J), dephosphorylate the 5 position of PI(3,4,5)P3 to produce PI(3,4)P2 (refs 11 , 12 ). Inositol polyphosphate 4-phosphatases, such as inositol polyphosphate 4-phosphatase type I (INPP4A), in turn dephosphorylate PI(3,4)P2 to produce PI(3)P, ultimately leading to termination of the PI3K/Akt signalling [13] . Mounting evidence has been provided to show that the PI3K/Akt signalling pathway is constitutively activated in a wide range of tumour types and is involved in tumour progression by promotion of uncontrolled cell proliferation, resistance to apoptosis and even distant metastasis [14] , [15] . Conversely, blockade of PI3K/Akt signalling has also been shown to markedly inhibit tumorigenicity and considered as a therapeutic approach in multiple types of cancer [16] , [17] , [18] . Aside from the mechanisms by which mutations or amplification of PI3K, RAS and epidermal growth factor receptor (EGFR) can lead to constitutively activated PI3K signalling, which confers poor prognosis in various types of human cancer, the functional loss of phosphoinositide phosphatases has also been demonstrated to be involved in initiation and progression of human cancers [19] , [20] , [21] , [22] . However, how cancer cells simultaneously override these negative regulations mediated by phosphoinositide phosphatases at diverse levels to exhibit constitutively activated PI3K/Akt remains largely unclear. By being able to simultaneously repress a variety of target genes through binding to their mRNA 3′-untranslated regions (3′UTRs), microRNAs (miRNAs) can potentially affect multiple steps of cancer progression and tumorigenesis [23] , [24] , [25] . Here, we show that our results together with public microarray data suggest that miR-508 is substantially overexpressed in clinical oesophageal squamous cell carcinoma (ESCC) and significantly correlated with poor patient prognosis. We demonstrate that miR-508 directly suppresses multiple phosphoinositide phosphatases, leading to constitutive activation of PI3K/Akt and inducing an aggressive phenotype of ESCC both in vitro and in vivo . Our findings uncover a novel regulatory and signalling pathway for the activation of PI3K/Akt signalling, thus supporting the clinical and functional significance of epigenetic events in cancer progression. Reduced INPP5J correlates with ESCC progression INPP5J, a member of the 5-phosphatase family, has been recently demonstrated to function as a vital negative regulator of PI3K/Akt signalling [12] , which is constitutively activated in numerous types of human cancers, including ESCC [26] . However, the clinical significance and biological role of INPP5J in ESCC remain unknown. Immunoblotting analysis indicated that expression of the INPP5J protein was differentially reduced in eight human ESCC samples paired with adjacent non-tumour tissues, as well as in 12 ESCC cell lines compared with two normal oesophageal epithelial cells (NEECs) ( Fig. 1a,b ). 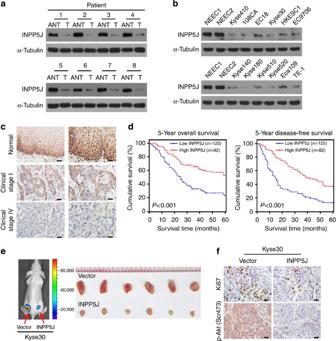Figure 1: Reduced INPP5J levels correlate with ESCC progression. (a,b) Western blotting analysis of INPP5J expression in eight pairs of ESCC samples (T) and adjacent normal tissues (ANT;a); and in two NEECs and 12 cultured ESCC cell lines (b). α-Tubulin served as the loading control. (c) IHC staining indicating that INPP5J protein expression is downregulated in human ESCC compared with normal oesophageal tissues. Clinical staging and clinicopathological TNM classification were determined according to the criteria proposed by International Union Against Cancer criteria. Immunohistochemical staining of INPP5J in representative samples of ESCC, and normal oesophageal tissues were shown. Scale bars, 50 μm (insets 20 μm). (d) Kaplan–Meier analysis of 5-year overall survival (left panel) or disease-free survival (right panel) curves for ESCC patients with low versus high expression of INPP5J (n=207;P<0.001). (e) Reconstitution of INPP5J inhibits ESCC tumorigenicity, as demonstrated by an ESCC tumour xenograft model. Left panel: representative images of tumour-bearing mice. Right panel: images of tumours from all mice in each group. (f) IHC staining detecting Ki67 and p-Akt (Ser 473) expression in the indicated tumours. Scale bars, 20 μm. Figure 1: Reduced INPP5J levels correlate with ESCC progression. ( a , b ) Western blotting analysis of INPP5J expression in eight pairs of ESCC samples (T) and adjacent normal tissues (ANT; a ); and in two NEECs and 12 cultured ESCC cell lines ( b ). α-Tubulin served as the loading control. ( c ) IHC staining indicating that INPP5J protein expression is downregulated in human ESCC compared with normal oesophageal tissues. Clinical staging and clinicopathological TNM classification were determined according to the criteria proposed by International Union Against Cancer criteria. Immunohistochemical staining of INPP5J in representative samples of ESCC, and normal oesophageal tissues were shown. Scale bars, 50 μm (insets 20 μm). ( d ) Kaplan–Meier analysis of 5-year overall survival (left panel) or disease-free survival (right panel) curves for ESCC patients with low versus high expression of INPP5J ( n =207; P <0.001). ( e ) Reconstitution of INPP5J inhibits ESCC tumorigenicity, as demonstrated by an ESCC tumour xenograft model. Left panel: representative images of tumour-bearing mice. Right panel: images of tumours from all mice in each group. ( f ) IHC staining detecting Ki67 and p-Akt (Ser 473) expression in the indicated tumours. Scale bars, 20 μm. Full size image To further investigate the expression status of INPP5J in ESCC, we conducted immunohistochemical staining for INPP5J in 207 ESCC patient specimens and 15 normal oesophageal tissue specimens. Immunohistochemistry (IHC) staining showed that INPP5J was strongly expressed in normal oesophageal tissues, but was slightly downregulated in low clinical stage and markedly repressed in high clinical stage ESCC samples ( Fig. 1c ). Moreover, statistical analysis revealed that INPP5J levels were inversely correlated with the clinical stage ( P =0.003) and the tumour-nodule-metastasis (TNM) classification (T: P <0.001; N: P =0.006; M: P =0.028) in patients with ESCC ( n =207; Supplementary Tables 1 and 2 ). Importantly, low INPP5J expression was found to be associated with shorter overall survival and poorer disease-free survival in primary ESCC ( P <0.001 and 0.001; Fig. 1d ). Taken together, these results suggest a possible link between reduced INPP5J and ESCC progression. To investigate the biological role of INPP5J in ESCC progression, the Kyse30 and Kyse510 ESCC cell lines were engineered to stably overexpress INPP5J ( Supplementary Fig. 1a ). As shown in Fig. 1e and Supplementary Fig. 1b,c , the tumours formed by INPP5J-transduced Kyse30 cells were smaller, in both size and weight, than the control tumours. Meanwhile, the expression of p-Akt (Ser 473) and Akt activity were markedly decreased in INPP5J-transduced tumours compared with those in vector control tumours ( Fig. 1f and Supplementary Fig. 1d ). Consistently, overexpressing INPP5J significantly decreased the proliferation rates and anchorage-independent growth abilities of ESCC cells, as well as the p-Akt level and Akt activity in ESCC cells ( Supplementary Fig. 2a–d ). Together, these results demonstrate that reconstitution of INPP5J inhibits ESCC tumorigenicity both in vivo and in vitro . miR-508 targets INPP5J However, no appreciable alteration of INPP5J mRNA expression was found in ESCC tissues compared with adjacent non-tumour tissues ( n =8; Supplementary Fig. 3a ), which is consistent with published microarray data (NCBI/GEO/GSE23400; n =106, including 53 non-tumour and 53 paired primary ESCC tissues; Supplementary Fig. 3b ), suggesting that the reduction of INPP5J in ESCC may be regulated at the post-transcriptional level. Analysis using publicly available algorithms (TargetScan and miRANDA) predicted INPP5J as a target of miR-508 ( Fig. 2a ), which is one of the most substantially overexpressed miRNAs in a published ESCC microarray data set (NCBI/GEO/GSE6188, n =257, including 104 non-tumour and 153 tumour samples) ( Fig. 2b ). In determining whether miR-508 affects INPP5J expression, we found that the expression of INPP5J protein was drastically decreased in miR-508-transduced ESCC cells and increased in cells transfected with the miR-508 antagomir ( Fig. 2c and Supplementary Fig. 4 ). Moreover, results of a luciferase reporter assay indicated that overexpression of miR-508 significantly repressed, whereas inhibition of endogenous miR-508 increased, the luciferase activity of INPP5J-3′UTR, and ectopically expressing miR-508 mutation had no inhibitory effect on the INPP5J-3′UTR luciferase activity ( Fig. 2d ). Taken together, these results demonstrate that INPP5J is a bona fide target of miR-508. 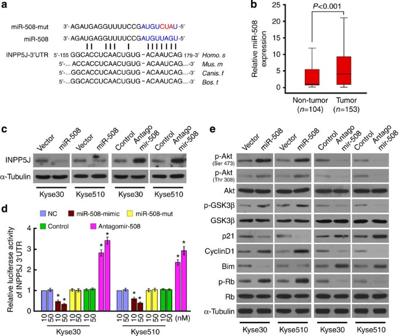Figure 2: miR-508 directly targets INPP5J and activates PI3K/Akt signalling. (a) Predicted miR-508 target sequences in the 3′UTR of INPP5J (INPP5J-3′UTR) and mutant containing three altered nucleotides in the seed sequence of miR-508 (miR-508-mut). (b) miR-508 was significantly overexpressed in ESCC analysed using published miaroarray data (NCBI/GEO/GSE6188,n=257, including 104 non-tumour and 153 tumour samples; boundaries of the boxes represent the lower and upper quartile. Lines within boxes and whiskers denote median and extremum, respectively.P<0.001;χ2-test). (c) Western blotting analysis of INPP5J expression in vector- or miR-508-transduced cells, or in cells transfected with negative control or miR-508 antagomir. α-Tubulin served as the loading control. (d) Luciferase assay of indicated cells transfected with the pGL3-INPP5J-3′UTR reporter with increasing amounts (10 and 50 nM) of negative control (NC), miR-508 mimic, control antagomir, miR-508 antagomir or miR-508-mut mimic. (e) Western blotting analysis of expression of p-Akt (Ser 473), p-Akt (Thr 308), Akt, p-GSK3β, GSK3β, p21, CyclinD1, Bim and pRb and p-pRb in the indicated cells. α-Tubulin served as the loading control. Each bar represents the mean±s.d. of three independent experiments. *P<0.05. Figure 2: miR-508 directly targets INPP5J and activates PI3K/Akt signalling. ( a ) Predicted miR-508 target sequences in the 3′UTR of INPP5J (INPP5J-3′UTR) and mutant containing three altered nucleotides in the seed sequence of miR-508 (miR-508-mut). ( b ) miR-508 was significantly overexpressed in ESCC analysed using published miaroarray data (NCBI/GEO/GSE6188, n =257, including 104 non-tumour and 153 tumour samples; boundaries of the boxes represent the lower and upper quartile. Lines within boxes and whiskers denote median and extremum, respectively. P <0.001; χ 2 -test). ( c ) Western blotting analysis of INPP5J expression in vector- or miR-508-transduced cells, or in cells transfected with negative control or miR-508 antagomir. α-Tubulin served as the loading control. ( d ) Luciferase assay of indicated cells transfected with the pGL3-INPP5J-3′UTR reporter with increasing amounts (10 and 50 nM) of negative control (NC), miR-508 mimic, control antagomir, miR-508 antagomir or miR-508-mut mimic. ( e ) Western blotting analysis of expression of p-Akt (Ser 473), p-Akt (Thr 308), Akt, p-GSK3β, GSK3β, p21, CyclinD1, Bim and pRb and p-pRb in the indicated cells. α-Tubulin served as the loading control. Each bar represents the mean±s.d. of three independent experiments. * P <0.05. Full size image miR-508 activates PI3K/Akt signalling Since INPP5J is a key negative regulator of PI3K/Akt signalling, we then investigated the effect of miR-508 on its downstream effectors. As shown in Fig. 2e , overexpressing miR-508 drastically increased, but silencing miR-508 decreased, the expression of p-Akt (Ser 473), p-GSK3β, CylinD1 and pRb. Concordantly, the expression of p21 and Bim decreased in miR-508-transduced ESCC cells and increased in miR-508-silenced cells ( Fig. 2e ). Therefore, our results indicate that miR-508 contributes to the activation of PI3K/Akt signalling. miR-508 directly targets phosphatase PTEN and INPP4A However, restoration of INPP5J expression in miR-508-transduced cells to the level comparable to that in control cells, via transfection with INPP5J ORF (without 3′UTR), only partially abrogated miR-508-induced Akt activity ( Fig. 3a ), suggesting that, in addition to INPP5J, other targets of miR-508 may also be involved in Akt activation. We found that phosphoinositide phosphatases PTEN and INPP4A are also potential targets of miR-508 ( Fig. 3b , upper panel). As expected, expression levels of PTEN and INPP4A were drastically reduced in miR-508-transduced cells but increased in miR-508 antagomir-transfected cells ( Fig. 3b , lower panel). Concordantly, overexpression of miR-508 decreased, and inhibition of miR-508 increased, the luciferase activity linked with the 3′UTR of these transcripts ( Fig. 3c ). However, ectopically expressing the miR-508 mutant did not result in repressive effects on their 3′UTRs ( Fig. 3c ). Importantly, results of the microribonucleoprotein (miRNP) immunoprecipitation assay showed that miR-508 selectively associated with INPP5J, PTEN and INPP4A, but not GAPDH ( Fig. 3d ), further confirming the specific effects of miR-508 on these targets. 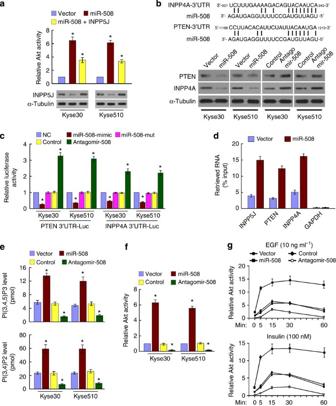Figure 3: miR-508 directly targets phosphoinositide phosphatase PTEN and INPP4A, and sustains phosphoinositide signalling. (a) Relative Akt activity (left panel) and INPP5J expression (right panel) in indicated cells. Recovery of INPP5J expression in miR-508-transduced cells comparable to that in control cells, via transfection with INPP5J ORF (without 3′UTR), only partially inhibited miR-508-induced Akt activity. (b) Upper panel: predicted miR-508 target sequence in PTEN-3′UTR and INPP4A-3′UTR. Lower panel: western blotting analysis of the expression of PTEN and INPP4A in the indicated cells. α-Tubulin served as the loading control. (c) Luciferase assay of indicated cells transfected with the pGL3-PTEN-3′UTR, pGL3-INPP4A-3′UTR reporter with miR-508 mimic, miR-508 antagomir or miR-508-mut mimic. (d) miRNP immunoprecipitation assay showed associations of miR-508 with INPP5J, PTEN and INPP4A.GAPDHserved as a negative control. (e) Detection of PI(3,4,5)P3 level (left panel) or PI(3,4)P2 (right panel) in miR-508-transduced cells or miR-508-inhibited cells compared with controls. (f) Relative Akt activity in miR-508-overexpressing or miR-508-inhibited ESCC cells compared with controls. (g) Relative Akt activity in the indicated cells, which were serum-starved and subsequently stimulated with EGF (10 ng ml−1, upper panel) or insulin (100 nM, lower panel) for indicated times. Each bar represents the mean±s.d. of three independent experiments. *P<0.05. Figure 3: miR-508 directly targets phosphoinositide phosphatase PTEN and INPP4A, and sustains phosphoinositide signalling. ( a ) Relative Akt activity (left panel) and INPP5J expression (right panel) in indicated cells. Recovery of INPP5J expression in miR-508-transduced cells comparable to that in control cells, via transfection with INPP5J ORF (without 3′UTR), only partially inhibited miR-508-induced Akt activity. ( b ) Upper panel: predicted miR-508 target sequence in PTEN-3′UTR and INPP4A-3′UTR. Lower panel: western blotting analysis of the expression of PTEN and INPP4A in the indicated cells. α-Tubulin served as the loading control. ( c ) Luciferase assay of indicated cells transfected with the pGL3-PTEN-3′UTR, pGL3-INPP4A-3′UTR reporter with miR-508 mimic, miR-508 antagomir or miR-508-mut mimic. ( d ) miRNP immunoprecipitation assay showed associations of miR-508 with INPP5J, PTEN and INPP4A. GAPDH served as a negative control. ( e ) Detection of PI(3,4,5)P3 level (left panel) or PI(3,4)P2 (right panel) in miR-508-transduced cells or miR-508-inhibited cells compared with controls. ( f ) Relative Akt activity in miR-508-overexpressing or miR-508-inhibited ESCC cells compared with controls. ( g ) Relative Akt activity in the indicated cells, which were serum-starved and subsequently stimulated with EGF (10 ng ml −1 , upper panel) or insulin (100 nM, lower panel) for indicated times. Each bar represents the mean±s.d. of three independent experiments. * P <0.05. Full size image miR-508 sustains phosphoinositide signalling Since the inhibitory effects of PTEN, INPP5J and INPP4A on PI3K/Akt signalling are associated with phosphoinositide metabolism, we then examined the effect of miR-508 on the production of PI(3,4,5)P3 and PI(3,4)P2. As shown in Fig. 3e , miR-508 overexpression significantly increased, but its inhibition decreased, the levels of PI (3,4,5) P3 and PI (3,4) P2 in ESCC cells. Consistently, the Akt activity was significantly induced in miR-508-transduced cells but decreased in miR-508 antagomir-transfected cells ( Fig. 3f ). Meanwhile, the strength and duration of p-Akt expression and Akt activity induced by epidermal growth factor (EGF) or insulin were markedly prolonged in miR-508-transduced cells and rapidly reduced in miR-508-silenced cells, whereas treatment with the PI3K inhibitor markedly inhibited the p-Akt expression and Akt activity induced by EGF or insulin in miR-508-overexpressing cells ( Fig. 3g and Supplementary Fig. 5a,b ), indicating that miR-508 overexpression sustains PI3K/Akt signalling in ESCC cells. Furthermore, we found that the PtdIns(3,4)P2 level markedly decreased in the miR-508-transduced cells in response to re-introduction of INPP4A, whereas silencing INPP4A increased the PtdIns(3,4)P2 level in the miR-508-inhibited cells ( Supplementary Fig. S6a ). In addition, individually silencing PTEN, INPP5J or INPP4A potently antagonized the repressive effect of the miR-508 antagomir on Akt activity ( Supplementary Fig. 6b ), demonstrating that PTEN, INPP5J and INPP4A are functionally relevant effectors of miR-508 in PI3K/Akt activation. Overexpression of miR-508 correlates with ESCC progression In agreement with the published ESCC miRNA microarray data (NCBI/GEO/GSE6188, n =257; Fig. 2b ), real-time PCR analysis revealed that miR-508 was markedly overexpressed in eight primary ESCC tissues compared with the paired tumour adjacent tissues, and in 12 tested ESCC cell lines as compared with two NEECs ( Fig. 4a,b ). Furthermore, statistical analysis revealed that miR-508 expression strongly correlated with the clinical stage ( P <0.001), TNM classification (T: P <0.001, N: P <0.001 and M: P <0.001) and histological differentiation ( P =0.002) in patients with ESCC ( Fig. 4c and Supplementary Table 3 ). Importantly, patients with higher miR-508 expression had a shorter survival time, whereas patients with lower miR-508 expression had a longer survival time ( P <0.001 and <0.001; Fig. 4d ). 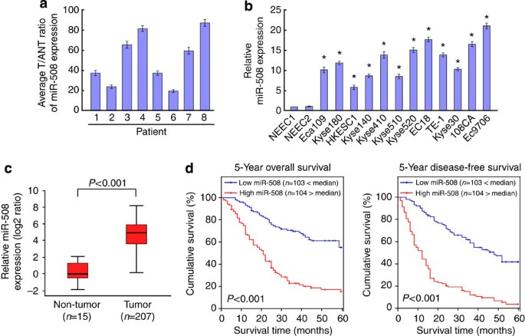Figure 4: Overexpression of miR-508 correlates with ESCC progression. (a,b) Real-time PCR analysis of miR-508 expression in eight pairs of ESCC samples (T) and adjacent normal tissues (ANT;a); and in two NEECs and 12 cultured ESCC cell lines (b). Transcript levels were normalized byU6expression. (c) miR-508 expression in 207 ESCC and 15 normal oesophageal tissues assessed by real-time PCR. Transcript levels were normalized byU6expression. Boundaries of the boxes represent the lower and upper quartile. Lines within boxes and whiskers denote median and extremum, respectively. (d) Kaplan–Meier analysis of 5-year overall (left panel) or disease-free (right panel) survival curves for ESCC patients with low miR-508 expression (< the median,n=103) or high miR-508 expression (> the median,n=104). Each bar represents the mean±s.d. of three independent experiments. *P<0.05. In addition, miR-508 expression was recognized as an independent prognostic factor ( P <0.001; Supplementary Table 4 ). Taken together, these results suggest that miR-508 overexpression has a role in human ESCC progression. Figure 4: Overexpression of miR-508 correlates with ESCC progression. ( a , b ) Real-time PCR analysis of miR-508 expression in eight pairs of ESCC samples (T) and adjacent normal tissues (ANT; a ); and in two NEECs and 12 cultured ESCC cell lines ( b ). Transcript levels were normalized by U6 expression. ( c ) miR-508 expression in 207 ESCC and 15 normal oesophageal tissues assessed by real-time PCR. Transcript levels were normalized by U6 expression. Boundaries of the boxes represent the lower and upper quartile. Lines within boxes and whiskers denote median and extremum, respectively. ( d ) Kaplan–Meier analysis of 5-year overall (left panel) or disease-free (right panel) survival curves for ESCC patients with low miR-508 expression (< the median, n =103) or high miR-508 expression (> the median, n =104). Each bar represents the mean±s.d. of three independent experiments. * P <0.05. Full size image miR-508 promotes ESCC aggressiveness in vitro and in vivo Next, we investigated the biological role of miR-508 overexpression in ESCC progression. As shown in Fig. 5a–c , overexpression of miR-508 markedly increased, whereas inhibition of miR-508 reduced, the proliferation rate, colony formation and anchorage-independent growth abilities of ESCC cells. Furthermore, overexpression of miR-508 rendered ESCC cells more resistant to chemotherapeutic agents, cisplatin and 5-fluorouracil, whereas inhibition of miR-508 sensitized the ESCC cells to these treatments ( Fig. 5d,e ). Meanwhile, the stimulatory effects of miR-508 on proliferation and survival of ESCC cells were drastically reduced upon treatment with an Akt inhibitor ( Fig. 5a–e ), demonstrating that functional Akt activation is vital to the biological effects of miR-508 in ESCC cells. 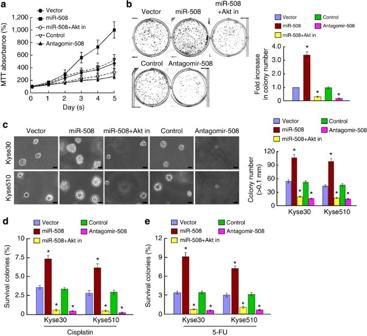Figure 5: miR-508 promotes ESCC cell proliferation and survivalin vitro. (a) Proliferation rate of the indicated ESCC cells examined with the MTT assay. (b) Representative images (left panel) and quantification (right panel) of indicated cells after crystal violet staining. (c) Representative micrographs (left panel) and quantification (right panel) of colonies determined by anchorage-independent growth assay. Scale bars, 100 μm. Colonies >0.1 mm in diameter were scored. (d,e) Survival percentage of colonies in the indicated cells treated with cisplatin (10 μM;d) or 5-fluorouracil (5-FU; 10 μM) for 36 h (e). Each bar represents the mean±s.d. of three independent experiments. *P<0.05. Figure 5: miR-508 promotes ESCC cell proliferation and survival in vitro . ( a ) Proliferation rate of the indicated ESCC cells examined with the MTT assay. ( b ) Representative images (left panel) and quantification (right panel) of indicated cells after crystal violet staining. ( c ) Representative micrographs (left panel) and quantification (right panel) of colonies determined by anchorage-independent growth assay. Scale bars, 100 μm. Colonies >0.1 mm in diameter were scored. ( d , e ) Survival percentage of colonies in the indicated cells treated with cisplatin (10 μM; d ) or 5-fluorouracil (5-FU; 10 μM) for 36 h ( e ). Each bar represents the mean±s.d. of three independent experiments. * P <0.05. Full size image The oncogenic role of miR-508 in ESCC progression was further examined using an in vivo tumour model. One group of mice was inoculated subcutaneously with Kyse30/vector cells in the left dorsal flank and with Kyse30/miR-508 cells in the right dorsal flank per mouse. As shown in Fig. 6a,b and Supplementary Fig. 7 , the tumours formed by miR-508-transduced cells were larger, in both size and weight, than the tumours formed from control cells. Another two groups were inoculated subcutaneously with Kyse30 cells in the left dorsal flank. Seven days later, the mice were then intratumorally injected with 100 μl of antagomir control or antagomir-508 (diluted in phosphate-buffered saline at 2 mg ml −1 ) three times per week for 2 weeks. Although the intratumorally injected antagomir control did not affect tumour development, injection of the miR-508 antagomir markedly inhibited tumour growth of ESCC cells. Consistently, the expression of p-Akt (Ser 473) and Akt activity were increased in miR-508-overexpressing tumours but downregulated in tumours injected with the miR-508 antagomir compared with control tumours ( Fig. 6c,d ). Meanwhile, miR-508-overexpressing tumours showed increased percentage of Ki67-positive cells and decreased TdT-mediated dUTP Nick-End Labeling (TUNEL)-positive cells, whereas miR-508-antagonized tumours displayed a lower Ki67 proliferation index and a higher percentage of TUNEL-positive apoptotic cells ( Fig. 6c ). These results demonstrate that miR-508 overexpression promotes ESCC tumorigenicity in vivo . 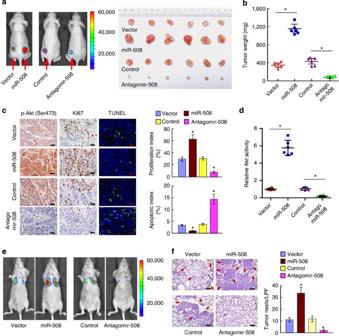Figure 6: Overexpression of miR-508 contributes to ESCC progressionin vivo. (a) Xenograft model in nude mice. Representative images of tumour-bearing mice (left panel) and images of tumours from all mice in each group (right panel). (b) Tumour weights in each group. (c) IHC staining showed that overexpression of miR-508 induced, whereas suppression of miR-508 inhibited, the proliferation and survival of ESCC cellsin vivo, as indicated by the expression of p-Akt and Ki67 and the numbers of TUNEL-positive cells. Scale bars, 20 μm. (d) Relative Akt activity in miR-508-overexpressing or miR-508-inhibited tumours compared with controls. (e) miR-508 overexpression significantly promoted, but miR-508 inhibition reduced, the tumour colonization and growth in the lung tissues. (f) Lung metastases in mice were confirmed by H&E staining. Arrows indicate the metastatic colonization of tumour cells in the lung tissues (left panel). The number of lung tumour nests in each group was counted under a low power field (LPF) and is presented as the mean+s.d. (right panel). Scale bars, 50 μm. Each bar represents the mean±s.d. of three independent experiments. *P<0.05. Figure 6: Overexpression of miR-508 contributes to ESCC progression in vivo . ( a ) Xenograft model in nude mice. Representative images of tumour-bearing mice (left panel) and images of tumours from all mice in each group (right panel). ( b ) Tumour weights in each group. ( c ) IHC staining showed that overexpression of miR-508 induced, whereas suppression of miR-508 inhibited, the proliferation and survival of ESCC cells in vivo , as indicated by the expression of p-Akt and Ki67 and the numbers of TUNEL-positive cells. Scale bars, 20 μm. ( d ) Relative Akt activity in miR-508-overexpressing or miR-508-inhibited tumours compared with controls. ( e ) miR-508 overexpression significantly promoted, but miR-508 inhibition reduced, the tumour colonization and growth in the lung tissues. ( f ) Lung metastases in mice were confirmed by H&E staining. Arrows indicate the metastatic colonization of tumour cells in the lung tissues (left panel). The number of lung tumour nests in each group was counted under a low power field (LPF) and is presented as the mean+s.d. (right panel). Scale bars, 50 μm. Each bar represents the mean±s.d. of three independent experiments. * P <0.05. Full size image Next, we examined the effect of miR-508 on ESCC progression in a lung colonization model. Nude mice were intravenously injected with miR-508-transduced cells and control cells via lateral tail veins. As shown in Fig. 6e–g , the number of tumour nests in the lungs formed by miR-508-transduced cells was significantly higher compared with control cells, indicating that miR-508 overexpression promotes ESCC cell lung colonization and growth. Meanwhile, 1 week after intravenous injections of Kyse30 cells in mice followed by a succession of either control antagomir or miR-508 antagomir treatments via the tail vein two times per week for 3 weeks, the miR-508 antagomir significantly reduced the lung colonization and growth compared with the control group ( Fig. 6c,f ). Clinical relevance of miR-508 and its targets in ESCC Finally, we examined whether miR-508-mediated suppression of INPP5J, PTEN and INPP4A, and Akt activity in ESCC are clinically relevant. IHC analysis revealed that the PTEN expression inversely correlated with ESCC grade and positively correlated with patient survival ( n =207; Fig. 7a , upper panel, and Supplementary Table 5 ), which was consistent with a previous report [27] . In the same cohort study, the INPP4A levels were also found to be correlated with patient survival time ( n =207; P <0.001) ( Fig. 7a , lower panel). Furthermore, we found that miR-508 expression inversely correlated with PTEN ( P <0.001), INPP5J ( P <0.001) and INPP4A levels ( P <0.001), but strongly correlated with p-Akt (Ser 473) expression ( P =0.004; Fig. 7b ). Moreover, using 10 freshly collected clinical ESCC samples of different clinical stages, miR-508 expression was shown to be inversely correlated with PTEN ( r =−0.718, P =0.011) and INPP5J ( r =−0.693, P =0.026) and INPP4A ( r =−0.663, P =0.037), but positively correlated with levels of p-Akt (Ser 473; r=0.724, P =0.006; Fig. 7c and Supplementary Fig. 8 ). Collectively, these results further support the notion that miR-508 overexpression activates PI3K/Akt signalling by repressing multiple phosphoinositide phosphatases, leading to ESCC progression and poor clinical outcomes ( Fig. 7d ). 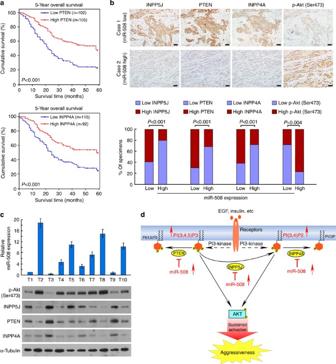Figure 7: Clinical relevance of miR-508 and expression of its targets in ESCC. (a) The Kaplan–Meier analysis of 5-year overall survival curves for ESCC patients with low versus high expression of PTEN (upper panel;n=207;P<0.001) or with low versus high expression of INPP4A (lower panel;n=207;P<0.001). (b) miR-508 levels were significantly associated with expression of INPP5J, PTEN, INPP4A and p-Akt (Ser 473) in 207 primary human ESCC specimens. Upper panel: two representative cases are shown. Scale bars, 50 μm. Lower panel: percentages of specimens showing low or high miR-508 expression relative to levels of INPP5J, PTEN, INPP4A and p-Akt (Ser 473). (c) Analysis of expression of miR-508 with the expression levels of INPP5J, PTEN, INPP4A and p-Akt (Ser 473) in 10 freshly collected human ESCC samples, including five clinical stage I-II and five clinical stage III-IV samples. (d) Proposed model. Upregulation of miR-508 represses multiple phosphoinositide phosphatases to sustain phosphoinositide signalling, leading to constitutive PI3K/Akt activation and ESCC aggressiveness. Figure 7: Clinical relevance of miR-508 and expression of its targets in ESCC. ( a ) The Kaplan–Meier analysis of 5-year overall survival curves for ESCC patients with low versus high expression of PTEN (upper panel; n =207; P <0.001) or with low versus high expression of INPP4A (lower panel; n =207; P <0.001). ( b ) miR-508 levels were significantly associated with expression of INPP5J, PTEN, INPP4A and p-Akt (Ser 473) in 207 primary human ESCC specimens. Upper panel: two representative cases are shown. Scale bars, 50 μm. Lower panel: percentages of specimens showing low or high miR-508 expression relative to levels of INPP5J, PTEN, INPP4A and p-Akt (Ser 473). ( c ) Analysis of expression of miR-508 with the expression levels of INPP5J, PTEN, INPP4A and p-Akt (Ser 473) in 10 freshly collected human ESCC samples, including five clinical stage I-II and five clinical stage III-IV samples. ( d ) Proposed model. Upregulation of miR-508 represses multiple phosphoinositide phosphatases to sustain phosphoinositide signalling, leading to constitutive PI3K/Akt activation and ESCC aggressiveness. Full size image Phosphoinositide signalling, a complex network cooperating by interconverting enzymes and phosphoinositides, has a crucial role in various cellular processes [1] , [2] , [3] . The phosphoinositide signalling can be activated by phosphorylation of phosphoinositides via phosphoinositide kinases, such as PI3K, and terminated by sequential dephosphorylation of phosphoinositides via phosphoinositide phosphatases, such as 3-phosphatase, 5-phosphatase and 4-phosphatase [5] , [28] . The oncogenic role of PI3K has been well established for the production of PI(3,4,5)P3 and PI(3,4)P2 levels, and constitutive activation of phosphoinositide signalling caused by mutations or amplification of EGFR, RAS and PI3K has been demonstrated to be involved in the initiation and progression of various types of human cancer, conferring poor prognosis [19] , [20] , [21] , [22] . However, how cancer cells concomitantly take priority over the negative regulation of the number of phosphoinositide phosphatases at diverse levels remains puzzling. Herein, we demonstrated that miR-508 is substantially overexpressed in ESCC and sustains PI3K/Akt signalling through enhancing PI(3,4,5)P3 and PI(3,4)P2 levels via directly suppressing multiple phosphoinositide phosphatases, including PTEN, INPP5J and INPP4A. Therefore, our findings reveal a novel mechanism that simultaneously disrupts the negative regulation by multiple phosphoinositide phosphatases, consequently resulting in constitutive PI3K/Akt activation in cancer cells. Over the past decade, phosphoinositide phosphatases have been emerging as important regulators of phosphoinositide signalling to balance the strength and duration of the PI3K/Akt cascade [29] . Deregulation of phosphoinositide phosphatases has been identified to largely contribute to the development and progression of cancers through constitutive activation of PI3K/Akt signalling [29] . For instance, the inositol 3-phosphatase PTEN is well demonstrated to be essential for prevention of tumorigenesis and functions as a vital tumour suppressor. PTEN is found to be commonly mutated or lost in numerous types of human cancers [30] , [31] , and monoallelic loss of PTEN is functionally haploinsufficient to facilitate tumour growth in the context of other somatic mutations [32] . INPP5J, an inositol 5-phosphatase recently identified, suppresses PI3K/Akt signalling by reducing the phosphorylation level of p-Akt (Ser 473) and was recently found to be downregulated in human melanoma, leading to promotion of cell proliferation and tumorigenicity in vivo [12] , [33] . Knockout of INPP4A was shown to sustain Akt activation and thereby promote cell proliferation, survival and tumorigenesis of mouse embryonic fibroblasts [13] , [34] . Hence, a better understanding of how these negative regulators are suppressed so that PI3K/Akt signalling is constitutively activated may provide new clues for the development of targeted cancer therapies. Our results and published microarray analysis (NCBI/GEO/GSE23400) show that the mRNA expression levels of PTEN, INPP4A and INPP5J are nearly the same in ESCC tissues as in paired non-tumour tissues ( Supplementary Fig. 9 ), suggesting that reduction of these phosphoinositide phosphatases in ESCC may be regulated at the post-transcriptional level. Interestingly, analysis using publicly available algorithms, a total of 12 genes associated with the regulation of phosphoinositide signalling, including PTEN, INPP4A, INPP5J, MINPP1, PLCXD3, IPMK, PI4KA, PI4K2A, AMG1, PIKFYVE, PIK3R5, PIK3R1 and PIK3C2G, were predicted as miR-508 potential targets. However, results from our serial experiments showed only PTEN, INPP4A and INPP5J as direct targets of miR-508 in ESCC. Importantly, individually silencing PTEN, INPP5J or INPP4A potently antagonized the repressive effect of the miR-508 antagomir on Akt activity, suggesting that the simultaneous repression of these three proteins may be necessary for the resultant oncogenic effects of miR-508. Despite therapeutic advances, current treatments for cancers remain challenging owing to their metastatic capacities. However, distant colonization of the metastasis cascade is highly rate limiting, and recent reports indicate that only a few metastatic cells with high tumour-initiating capacity respond to the local microenvironment by proliferating [35] . Therefore, inhibition of the growth at secondary sites represents a potential therapeutic strategy for cancer metastasis [36] , [37] . As the PI3K/Akt pathway is well known to confer survival advantage in cancers by inducing uncontrolled cell proliferation, chemo-resistance and metastasis, it has been considered an important therapeutic target for cancers [17] , [18] . Thus, a better understanding of the molecular mechanisms underlying PI3K/Akt activation in ESCC may facilitate the identification of novel therapeutic targets for ESCC. Here, we report that Akt activity can be robustly activated by miR-508 overexpression but inhibited by antagonizing endogenous miR-508 in ESCC. Meanwhile, overexpression of miR-508 markedly promotes, whereas inhibition of miR-508 impairs, ESCC cell proliferation and survival both in vitro and in vivo . Notably, using a lung colonization model, we found that overexpressing miR-508 increases, but intravenous injections of miR-508 antagomir treatments significantly decreases, the tumour cell colonization and growth in the lungs, suggesting an effective role of miR-508 antagomir in the inhibition of distantly colonizing metastatic cells. Therefore, our results suggest that miR-508 exerts an oncogenic role in ESCC progression, and its inhibition may also allow development of a novel therapeutic strategy. In summary, our study reveals that miR-508 overexpression has an important role in ESCC progression and that miR-508 is a critical activator of PI3K/Akt signalling. Understanding the precise role of miR-508 in the pathogenesis of ESCC and activation of the PI3K/Akt signalling pathway will increase our knowledge of the biological basis of cancer progression and may also allow the development of new therapeutic strategies against ESCC. Cell lines and cell culture Primary cultures of NEECs were established from fresh specimens of adjacent noncancerous oesophageal tissue >5 cm from the cancerous tissue [38] . The ESCC cell lines KYSE30, KYSE140, KYSE180, KYSE410, KYSE510 and KYSE520 were obtained from Deutsche Sammlung von Mikroorganismen und Zellkulturen, the German Resource Centre for Biological Material [39] . All cell lines were authenticated by short tandem repeat fingerprinting at Medicine Lab of Forensic Medicine Department of Sun Yat-Sen University (Guangzhou, China). Tissue specimens and clinicopathological characteristics The total 207 paraffin-embedded, archived ESCC samples used in this study were histopathologically and clinically diagnosed at the Sun Yat-sen University Cancer Center between 2003 and 2009. Clinical staging and clinicopathological TNM classification were determined according to the criteria proposed by International Union Against Cancer criteria. Written informed consent was obtained from all patients before the study. The use of the clinical specimens for research purposes was approved by the Institutional Research Ethics Committee. The clinicopathological characteristics of the samples are summarized in Supplementary Table 1 . Eight freshly collected ESCC tissues and matched adjacent non-tumour oesophageal tissues from the same patient were frozen and stored in liquid nitrogen until required. Immunohistochemistry IHC analysis was performed on the 207 paraffin-embedded ESCC tissue sections [40] , using the following primary antibodies, anti-INPP5J antibody (1:100; Proteintech, WuHan, China), anti-p-Akt (Ser 473;1:50), anti-Ki67 (1:200), anti-PTEN (1:100) antibodies (Cell Signaling, Danvers, MA, USA), anti-INPP4A antibody (1:100; Abcam, Cambridge, MA, USA). The degree of immunostaining of formalin-fixed, paraffin-embedded sections were reviewed and scored separately by two independent pathologists. The scores were determined by combining the proportion of positively stained tumour or NEECs and the intensity of staining. Cell proportions were scored as follows: 0, no positive cells; 1, <10% positive cells; 2, 10–35% positive cells; 3, 35–75% positive cells; and 4, >75% positive cells. Staining intensity was graded according to the following standard: 1, no staining; 2, weak staining (light yellow); 3, moderate staining (yellow brown); and 4, strong staining (brown). The staining index (SI) was calculated as the product of the staining intensity score and the proportion of positive cells. Using this method of assessment, we evaluated protein expression in benign oesophageal epithelia and malignant lesions by determining the SI, with possible scores of 0, 2, 3, 4, 6, 8, 9, 12 and 16. Samples with a SI ⩾ 8 were determined as high expression and samples with a SI <8 were determined as low expression. Cutoff values were determined on the basis of a measure of heterogeneity using the log-rank test with respect to overall survival. Xenografted tumour model, IHC and H&E staining BALB/c-nu mice (5–6 weeks of age, 18–20 g) were purchased from the Center of Experimental Animal of Guangzhou University of Chinese Medicine, and were housed in barrier facilities on a 12-h light/dark cycle. All experimental procedures were approved by the Institutional Animal Care and Use Committee of Sun Yat-sen University. The BALB/c nude mice were randomly divided into groups ( n =6 per group). One group of mice was inoculated subcutaneously with Kyse30/vector cells (5 × 10 6 ) in the left dorsal flank and with Kyse30/miR-508 cells (5 × 10 6 ) in the right dorsal flank per mouse. Another two groups were inoculated subcutaneously per mouse with Kyse30 cells (5 × 10 6 ) in the left dorsal flank. Seven days later, the mice were then intratumorally injected with 100 μl of antagomir control or antagomir-508 (diluted in phosphate-buffered saline at 2 mg ml −1 ) three times per week for 2 weeks. Tumours were examined twice weekly; length, width and thickness measurements were obtained with calipers, and tumour volumes were calculated. Tumour volume was calculated using the equation (L × W 2 )/2. On day 40, tumours were detected by an IVIS imagining system (Caliper), then animals were euthanized, tumours were excised, weighed and paraffin embedded. Serial 6.0 μm sections were cut and subjected to immunohistochemical and haematoxylin and eosin (H&E) staining. After deparaffinization, sections were IHC analysed using an anti-Ki67 (Dako, Glostrup, Denmark), anti-p-Akt antibody (Cell Signaling) or H&E stained with Mayer’s haematoxylin solution. Proliferation index was quantized by counting proportion of Ki67-positive cells. Apoptotic index was measured by percentage of TUNEL-positive cells. The effect of miR-508 on ESCC progression was further examined in a lung colonization model. Two groups were intravenously injected with miR-508-transduced cells and control cells via lateral tail veins. Another two groups were intravenously injected with Kyse30 cells in the mice, followed by a succession of either control antagomir or antagomir-508 treatments via the tail vein, two times per week for 3 weeks. Tumour colonization and growth in the lung tissues were detected by an IVIS imagining system (Caliper). Mice were killed 40 days after injection. Lungs were fixed in formalin and embedded in paraffin using the routine method. H&E staining was performed on sections from paraffin-embedded samples for histological evidence of the tumour phenotype. The number of lung tumour nests in each group was counted under a low power field and is presented as the mean+s.d., * P <0.05. Western blotting analysis Western blotting was performed using the primary antibodies, anti-p-Akt (1:500; Ser 473), anti-p-Akt (1:500; Thr 308), anti-Akt (1:1,000), anti-p-GSK3β (1:500), anti-GSK3β (1:1,000), anti-CyclinD1 (1:1,000), anti-Bim (1:1,000), anti-p21 (1:500), anti-pRb (1:1,000), anti-Rb (1:1,000), anti-PTEN (1:1,000) antibodies (Cell Signaling), anti-INPP4A antibody (1:500; Abcam) and anti-INPP5J antibody (1:500; Proteintech). Following the initial western blot assay, the membranes were stripped and re-probed with anti-α-tubulin (1:500; Sigma, St Louis, MO, USA) as a protein loading control. Mimic, antagomir, plasmids and virus constructs miR-508 mimic and antagomir-508 were purchased from RIBOBIO company (GuangZhou, China). Human INPP5J and miR-508 genes were amplified by PCR and cloned into the pMSCV-puro-retro vector. Transfection of small interfering RNAs (siRNAs) or plasmids was performed using Lipofectamine 2000 reagent (Invitrogen, Carlsbad, CA, USA) according to the manufacturer’s instructions. Stable cell lines expressing INPP5J and miR-508 were generated by retroviral infection using HEK293T cells, and selected with 0.5 μg ml −1 puromycin for 10 days. Colony formation assays Cells were plated in six-well plates (5 × 10 2 cells per plate) and cultured for 10 days. The colonies were stained with 1% crystal violet for 30 s after fixation with 10% formaldehyde for 5 min. Cell treatments Akt inhibitor MK-2206 (1 μM; Selleck Chemicals, Houston, TX, USA), PI3K inhibitor LY294002 (10 μM; EMD Millipore, Billerica, MA, USA) or 5-fluorouracil (10 μM; Sigma) was dissolved in dimethyl sulphoxide, and cisplatin (10 μM; Sigma) was dissolved in 0.9% NaCl. RNA extraction and real-time quantitative PCR Total miRNA from cultured cells and ESCC tissue samples was extracted using the mirVana miRNA Isolation Kit (Ambion, Austin, TX, USA) according to the manufacturer’s manual. The expression level of miR-508 was quantified using miRNA-specific TaqMan MiRNA Assay Kit (Applied Biosystems). Real-time PCR was performed using the Applied Biosystems 7,900 Sequence Detection system. The expression of miRNA was defined based on the threshold cycle ( C t ), and relative expression levels were calculated as 2 −[( C t of miR-508)−( C t of U6)] after normalization with reference to the quantification of U6 small nuclear RNA expression. Primers and oligonucleotides Cloning miR-508: 5′-GCCGGATCCAGAAAGTCCAGGG CTGAGAAG-3′ and 5′-GCCACTAGTTTTGGTGCAGAGGGATGCT-3′; cloning INPP5J ORF: 5′-GCCGAATTCATGGAGGGCCAGAGCAGCAG-3′ and 5′-GCCACTAGTTCAGGGCCCCAGGCCCCCTT-3′; cloning INPP5J-3′UTR-luc: 5′-GCCCCGCGGGTGGGG TAG GCAGATGGG-3′ and 5′-GCCCTGCAGTGACCTCCAGGATTGGGAC-3′; cloning PTEN -3′UTR-luc: 5′-GCCCCGCGGAACAAAGAATGGGCTTGAAACA-3′ and 5′-GCCCTGCAGGGGGAGCACTATGAAGAAATGA-3′; cloning INPP4A-3′UTR-luc: 5′-GCCCCGC GGC CCTTTAGCCTGTCTCCTGTT-3′ and 5′-GCCCTGCAGCACCC TACCTGATGCCCAC-3′; GAPDH primers for RIP: 5′-TCCCCCACCACACTGAATCT-3′ and 5′-GCCCCTCCCCTCT TCAAG-3′; INPP5J primers for RIP: 5′-CATTCTGCCTCAATCTTTTGC-3′ and 5′-GACC CCAGTTGTCCACCC-3′; PTEN primers for RIP: 5′-GGCCGCTGTCACTGCTTG-3′ and 5′-ACCCCAATACAGATTCACTTCC-3′; INPP4A primers for RIP: 5′-TGGGGAG GACTG CTTA TTGG-3′ and 5′-TGCTGACTTCTGAGTAGGAGGG-3′; INPP5J primers for real-time PCR: 5′-ACACAGTCAGCGACCACAAG-3′ and 5′-CACTCATCTGCCACC TCCA-3′; INPP5J siRNA: 5′-ACGAUAC CAGUGCCAAGAAAC-3′; PTEN siRNA: 5′-CCACAAAUGAAGGGAUAUAAA-3′; INPP4A siRNA: 5′-GAUGAGUGACAAGGCCAAGAA-3′. miRNP immunoprecipitation Cells were co-transfected with HA-Ago1 together with 100 nM miR-508, followed by HA-Ago1 immunoprecipitation using HA-antibody. Real-time PCR analysis of the IP material was used to test the association of the mRNA of INPP5J, PTEN and INPP4A with the RNA-induced silencing complex (RISC) complex. Akt activity assay Cells were serum-starved and treated with EGF (10 ng ml −1 ) or insulin (100 nM) for 5 min. To measure kinase activities of in cells or tumour tissues, Akt was precipitated by a specific anti-Akt antibody. The immune complexes were then incubated with a biotinylated peptide substrate that became phosphorylated in the presence of activated Akt. The phosphorylated substrates, which reflected the activity of Akt kinase in the extract, was then quantified with the K-LISA Akt Activity Kit (Calbiochem, Darmstadt, Germany) that comprises a primary antibody recognizing the phosphorylated substrate peptides. Luciferase assay Ten thousand cells were seeded in triplicate in 48-well plates and allowed to settle for 24 h. One hundred nanograms of luciferase reporter plasmids or the control luciferase plasmid, plus 5 ng of pRL-TK renilla plasmid (Promega, Madison, WI, USA), were transfected into ESCC cells using the Lipofectamine 2000 reagent (Invitrogen) according to the manufacturer’s recommendation. Luciferase and renilla signals were measured 24 h after transfection using the Dual Luciferase Reporter Assay Kit (Promega) according to a protocol provided by the manufacturer. Three independent experiments were performed, and the data are presented as mean±s.d. Analysis of phosphoinositide levels Cells were serum-starved and treated with EGF (10 ng ml −1 ) for 5 min. Phosphoinositides were extracted from cells and subjected to enzyme-linked immunosorbent assay (ELISA) assay using a PI(3,4,5)P3 or PI(3,4)P2 mass ELISA kit (Echelon, Salt Lake City, UT, USA). Briefly, lipids were extracted with 2.25 ml of MeOH, CHCl 3 , 12 M HCl (80:40:1) for 15 min at room temperature and partitioned by centrifugation after the addition of 0.75 ml of CHCl 3 and 1.35 ml of 0.1 M HCl. The lower phase was vacuum-dried and dissolved in appropriate buffers. Phosphoinositide samples and standards were then applied for the ELISA assay according to the supplier’s instructions. The reaction was terminated by adding stop solution (0.5 M H 2 SO 4 ), and the absorbance was measured at 450 nm. Experiments were repeated twice, and all samples were run in triplicate per experiment. Data are presented as mean±s.d., and statistical significance was assessed by two-tailed, paired Student’s t -test. Statistical analysis All statistical analyses were carried out using SPSS13.0 statistical software. The χ 2 -test was used to analyse the relationship between miR-508 and targets expression. Survival curves were plotted using the Kaplan–Meier method and compared by log-rank test. Survival data were evaluated by univariate and multivariate Cox regression analyses. P <0.05 was considered statistically significant. How to cite this article: Lin, C. et al . miR-508 sustains phosphoinositide signalling and promotes aggressive phenotype of oesophageal squamous cell carcinoma. Nat. Commun. 5:4620 doi: 10.1038/ncomms5620 (2014).